Water induced ultrathin Mo2C nanosheets with high-density grain boundaries for enhanced hydrogen evolution Grain boundary controlling is an effective approach for manipulating the electronic structure of electrocatalysts to improve their hydrogen evolution reaction performance. However, probing the direct effect of grain boundaries as highly active catalytic hot spots is very challenging. Herein, we demonstrate a general water-assisted carbothermal reaction strategy for the construction of ultrathin Mo 2 C nanosheets with high-density grain boundaries supported on N-doped graphene. The polycrystalline Mo 2 C nanosheets are connected with N-doped graphene through Mo–C bonds, which affords an ultra-high density of active sites, giving excellent hydrogen evolution activity and superior electrocatalytic stability. Theoretical calculations reveal that the d z 2 orbital energy level of Mo atoms is controlled by the MoC 3 pyramid configuration, which plays a vital role in governing the hydrogen evolution activity. The d z 2 orbital energy level of metal atoms exhibits an intrinsic relationship with the catalyst activity and is regarded as a descriptor for predicting the hydrogen evolution activity. Owing to the high gravimetric specific energy density and environmentally friendly characteristics, hydrogen energy has emerged as one of the most promising alternatives to fossil fuels [1] , [2] . Electrochemical hydrogen evolution reaction (HER) provides an attractive way for efficient H 2 production from water electrolysis, in which catalysts are critical for developing renewable energy conversion technologies [3] . To date, platinum (Pt)-based materials are considered to be the most active HER catalysts, but the scarcity and high cost of Pt rigorously hamper their widespread applications [4] . Therefore, developing earth-abundant alternatives to Pt-based catalysts for achieving efficient H 2 generation is highly desirable. Molybdenum carbide (Mo 2 C), an excellent early transition-metal carbide, has intensely awakened ever-growing interest as a promising HER electrocatalyst because its electronic structure is virtually analogous to that of Pt metal [5] , [6] . Nevertheless, Mo 2 C surface shows excessively strong Mo–H binding energy, which hinders the desorption of adsorbed H to generate H 2 , severely deteriorating the electrochemical HER activity [7] . Grain boundaries (GBs), as a type of planar defect, are effective to directly tune the surface atomic and electronic structure, significantly altering the intrinsic reactivity of nanocrystalline materials [8] , [9] . Specifically, GBs create lattice distortion regions in Mo 2 C polycrystals by stabilizing dislocations, which could provide an optimized electronic structure for tailoring the binding energy of Mo–H, consequently accelerating the H 2 production. However, conventional bulk materials are typically limited to the surface GB density, which is not available for practical catalytic reactions due to the relatively low accessibility of active sites. Compared with bulk counterparts, ultrathin two-dimensional (2D) nanostructures possess sufficient interplanar active sites and shorter reactant/product diffusion length, and have been intensively reported as promising candidates for HER [10] . Currently, most of the Mo 2 C nanostructures are synthesized from either high-temperature carburization of costly/toxic molybdenum precursors (e.g., Mo foil, MoF 6 , and Mo(CO) 6 ) with carbonaceous gases (e.g., CH 4 , C 2 H 6 , and CO) [7] , [11] or the selectively etching layered ternary Mo-containing phases [12] , [13] . Nevertheless, in the former method, the resultant carbide surface generally suffers from severe char contamination from the pyrolysis of carbonaceous gases, inhibiting the exposure of active sites; in the latter, the delamination yield and defect controllability of Mo 2 C sheets derived in aqueous fluoride-containing acidic solutions are not satisfactory. In this context, nearly all the above-mentioned methods can only introduce small changes in the structural and chemical configuration of Mo 2 C catalysts, resulting in poor tunability for altering the catalytic performance. Therefore, a facile approach for developing high-density and fully exposed GBs on ultrathin 2D Mo 2 C nanostructure is highly desired. Herein, we propose an effective strategy to achieve ultrathin Mo 2 C nanosheets (NSs) with rich GBs supported on N-doped graphene (H-Mo 2 C/NG) via hydrothermal and water-assisted carbothermal reactions. During the carbonization process, water induces the structural evolution of Mo 2 C nanocrystals from nanoparticles (NPs) to NSs and controls the GB density of Mo 2 C NSs as well. The high-density GBs in Mo 2 C NSs provide an ultra-high fraction of active sites, significantly improving the inherent HER activity of H-Mo 2 C/NG. Theoretical calculations show that the GBs in Mo 2 C NSs modulate the configuration of MoC 3 pyramid, which thereby regulates the Mo d z 2 orbital energy level, manipulating the Mo–H bond strength of H-Mo 2 C/NG catalyst and influencing the HER activity. This work opens up an avenue for the development of high-efficiency catalysts through GB engineering. Controllable construction of ultrathin Mo 2 C NSs with high-density GBs Mo 2 C NSs supported on N-doped graphene (NG) were constructed in situ by facile hydrothermal and water-assisted carbothermal reactions (Fig. 1a ). Typically, graphene oxide (GO) and (NH 4 ) 6 Mo 7 O 24 ·4H 2 O were dissolved into deionized water and then the homogeneous solution was subjected to a hydrothermal reaction to obtain a homogeneous mixture composed of amorphous MoO 3 supported on reduced GO sheets (MoO 3 /RGO) (Supplementary Fig. 1 ) [7] . Next, the mixture was freeze-dried and then treated at 800 °C under NH 3 /Ar gas. Finally, only Mo 2 C NPs decorated on NG were obtained when the MoO 3 /RGO intermediate was water-free. However, when MoO 3 /RGO intermediate contained sufficient water concentration (18.56 wt%), Mo 2 C NSs with high-density GBs were constructed in situ and anchored on NG. Further details of the experiments were provided in Methods. Fig. 1: Formation of H-Mo 2 C/NG. a Schematic diagram of the synthesis of Mo 2 C/NG and H-Mo 2 C/NG. b Various reaction states of IS NP and IS NS along the reaction pathway. Inset shows the corresponding reaction Δ H diagram. The reaction Δ H for TS NS conversion to TS NS -C (–2.48 eV) is lower than that of TS NP conversion to TS NP -C (–0.73 eV), indicating that water promotes the formation of Mo 2 C during carbonization process. Full size image To illustrate the growth behavior of Mo 2 C nanocrystals with the assistance of water, density functional theory (DFT) calculations were performed. As shown in Fig. 1b , two theoretical model systems consisting of initial MoO 3 without H 2 O (IS NP ) and with H 2 O (IS NS ) are constructed, and the structural evolution mechanisms of Mo 2 C products are discussed from a reaction enthalpy (Δ H ) viewpoint. During the carbonization process, IS NP and IS NS first absorb heat and dissociate into transition states of TS NP and TS NS , respectively, and they then react with C atoms in RGO to form Mo 2 C. Generally, RGO has two types of C atoms, namely, the highly reactive carbon at the edge and the relatively inertness carbon of the six-membered C-ring far away from the edge [14] . Because H-bonded graphene has a structure analogous to benzene (Ph), the chemical properties of the compounds can be thought to be similar [15] . For simplicity, the C atoms extracted from the edge of the graphene lattice, as well as the free Ph radicals, react with TS NP and TS NS to produce TS NP -C, TS NP -Ph, TS NS -C, and TS NS -Ph, respectively. Of course, these model structures are much simpler than those in the actual experiment, yet, they are sufficient to study the interaction between two substances. Theoretical calculations show that Δ H values for TS NP and TS NS reacting with C atoms are both negative, which indicates that the C atoms from RGO can carbonize MoO 3 to form Mo 2 C. In anhydrous atmosphere, C atoms are chemically intercalated into common MoO 3 motifs, reducing MoO 3 into Mo 2 C NPs decorated on defective NG. In addition, the reaction Δ H of TS NP to produce TS NP -Ph is 0.45 eV, suggesting that TS NP fails chemically bind with the six-membered C-ring. But the reaction Δ H for TS NS to produce TS NS -Ph is –1.45 eV, which indicates that TS NS tends to combine with six-membered C-ring on RGO basal plane, thus inducing the lateral arrangement of Mo 2 C lattice along 2D direction [16] . In general, common MoO 3 without H 2 O can only react with carbon on RGO edge, producing Mo 2 C NPs. While MoO 3 with H 2 O not only reacts with the edge C atoms but also readily combines with six-membered C-ring along the RGO basal plane; in this situation, epitaxial growth is carried out to enlarge the Mo 2 C domain, achieving a coalesced NSs with several micrometers in lateral size. Especially, in the presence of H 2 O, due to the guest–host interaction between H 2 O and MoO 3 [17] , a unique Mo–O configuration is obtained and anchored on RGO, which serves as the nucleation site for Mo 2 C growth. As the activated carbon species encounter the Mo–O configuration, the dense seeds begin to individually nucleate at multiple regions. Consequently, these simultaneously grown nanocrystals merge together seamlessly and eventually form multi-faceted Mo 2 C NSs, which thereby hinders the growth of Mo 2 C grains in the radial orientation, leaving behind numerous GBs. In this situation, the RGO intermediate not only provides C source for Mo 2 C growth, but also acts as a robust supports for Mo 2 C nanodomains to nucleate and finally splice into NSs; in turn, the formed Mo 2 C NSs are covalently connected with underneath NG sheets through Mo–C bonds, which ensures the high inherent stability of Mo 2 C hybrids. Morphologies and structures of the Mo 2 C hybrids were characterized with atomic force microscopy (AFM), transmission electron microscopy (TEM), and high-angle annular dark-field scanning TEM (HAADF-STEM) measurements. For Mo 2 C/NG, Fig. 2a, b and Supplementary Fig. 2 show that high-density and discrete Mo 2 C NPs (diameter <5 nm) are uniformly loaded on NG layers. In contrast, in H-Mo 2 C/NG, GB-rich Mo 2 C NSs with a uniform thickness of ~1.0 nm, corresponding to 2 ~ 3 layers of unit cells, are well-distributed on NG (Fig. 2c, d and Supplementary Figs. 3 , 4 ), affording a very high proportion of exposed active sites. Procession electron diffraction (PED) measurements under TEM were employed to collect orientation maps and extract GB density. As shown in Fig. 2e and Supplementary Fig. 5 , the crystallographic orientations of each grain in the polycrystalline microstructure are random, and especially abundant intersections between domain walls can be observed. The GB density of Mo 2 C NSs in Mo 2 C hybrids is summarized in Supplementary Fig. 6 , where the statistical region of each sample is ~ 20,000 nm 2 . Obviously, H-Mo 2 C/NG possesses the highest GB density of 138 ± 3 μm −1 , clearly demonstrating that the water content in MoO 3 /RGO effectively manipulates the GB density of Mo 2 C NSs, consistent with TEM results (Supplementary Figs. 7 – 9 and Supplementary Note 1 ). It is worth mentioning that the supply of NH 3 (Supplementary Fig. 10 and Supplementary Note 2 ) and the sufficient oxygen-containing functional groups on GO surface (Supplementary Figs. 11 – 14 and Supplementary Note 3 ) are necessary for the formation of GB-rich Mo 2 C NSs. Furthermore, tens of HAADF-STEM images clearly reveal that Mo 2 C NSs composed of individual grains with nanometer size (Fig. 2f and Supplementary Fig. 15 ), which forms chemically connected interfaces with numerous GBs and triple junctions, indicating full exposure of high-density active sites in electrocatalysis. Fig. 2: Structural characterization of Mo 2 C hybrids. a , c AFM images of a Mo 2 C/NG and c H-Mo 2 C/NG and their corresponding height profiles. b , d TEM images of b Mo 2 C/NG and d H-Mo 2 C/NG. Mo 2 C NPs are highlighted by yellow dotted circles. e Inverse pole figure (IPF) images from PED analysis of H-Mo 2 C/NG. f Representative HADDF-STEM image of H-Mo 2 C/NG, the dashed lines point out the irregular GBs. Full size image Atomic structure of GBs on Mo 2 C NSs in H-Mo 2 C/NG We employed HAADF-STEM characterization to examine the atomic structure of GBs. The inspection of dozens of boundary locations systematically found that the nanocrystalline grains in Mo 2 C NSs are seamlessly stitched with irregular GBs (Fig. 3 and Supplementary Fig. 16 ). Figures 3a, a1–a3 obviously display that two Mo 2 C nanograins form a corrugated GB with an angle of 15°, as well as stacking faults (SFs) and off-centered Mo columns. Furthermore, a conspicuous strain concentration is discovered in the vicinity of the GB (Fig. 3b ). Compressive strain (–0.136 ± 0.036) and tensile strain (0.801 ± 0.484 and 0.107 ± 0.086) coexist (Supplementary Fig. 17 ), ensuring that the average strain of Mo 2 C NSs almost offsets. In addition, Fig. 3c demonstrates sharp GBs in the same specimen, offering an alternative view. The atomic structure of Mo 2 C NS is directly determined by characterizing the nanostructure along two zone axes, where two Z-contrast images closely resemble the structural projection of hexagonal close-packed (hcp) Mo 2 C, and their fast Fourier transform (FFT) patterns can be well indexed by hcp cells along their [1 \(\overline{2}\) 1 \(\overline{3}\) ] h and [01 \(\overline{1}\) 1] h directions, respectively (Fig. 3c1, c2 ). Where misorientation angle (38°), step dislocations, and terraced step edges are observed (Fig. 3c3, c4 ). Particularly, the misorientation angle distribution of observed adjacent grains reveals that the misorientation angle of GBs mostly ranges from 18° to 39° (Supplementary Fig. 18 ). High-angle GBs are the dominant type of planar defects in all of the Mo 2 C NSs examined, distinguishing from conventional Mo 2 C nanocrystals grown on graphene without water involved, where low-angle GBs predominate [18] . Compared with low-angle GBs, high-angle irregular GBs have a greater degree of atomic disorder, which generates a suitable electronic structure [19] , so as to optimize the H adsorption behavior. Impressively, Mo 2 C NSs also occur a topotactic transition from a conventional phase of hcp to a metastable phase of face-centred cubic (fcc), which highlights the controlled synthesis of Mo 2 C NSs with unconventional crystal phases through water-assisted carbonization process. Figure 3d, e and Supplementary Fig. 19 show representative HAADF-STEM images of fcc/hcp GB superstructures. 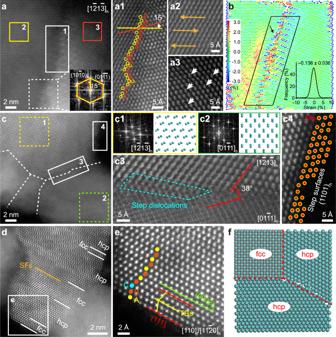Fig. 3: Local atomic structure of GBs on Mo2C NSs in H-Mo2C/NG. aA tilted GB in Mo2C NS. Inset of the FFT pattern indicates a 15° misorientation between grains.a1Enlarged HAADF-STEM image of region 1 ina. Yellow and tangerine circles represent the Mo atoms on the left and right sides of GB, respectively.a2,a3Enlarged HAADF-STEM images of regions 2 and 3 ina. The orange and white arrows represent SFs and displacements, respectively.bLattice shear distortion determined from panela, analyzed using the lattice distortion analysis (LADIA) programme. Inset is the quantitative distribution of shear strain for atoms in black-boxed region. The arrow indicates the direction of strain. The strains near GBs range from –5% to 5%. The atoms are colored according to strain scale, that is, colors for positive values represent tensile strain and those for negative values represent compressive strain.cThe hcp/hcp lattices along the [1\(\overline{2}\)1\(\overline{3}\)]h/[01\(\overline{1}\)1]hdirection, the white dashed lines point out the irregular GBs.c1,c2FFT patterns taken from regions 1 and 2 inc, and the corresponding projected supercell models of hcp Mo2C. The cyan balls represent Mo atoms.c3,c4Enlarged HAADF-STEM images of regions 3 and 4 incdisplaying tilt GBs, step dislocations, and stepped surfaces. Step dislocations, caused by the insertion of additional planes into the otherwise self-contained lattice, highlighted with the cyan dotted box. The atomic displacement arose from this distortion at GBs is usually much greater than the relaxation displacement occurring on the crystal surface as well as the displacement caused by the coherent strain through epitaxial thin-film growth18.dThe fcc/hcp lattices along the [110]f/[11\(\overline{2}\)0]hdirection. The fcc/hcp GBs are marked with white solid lines.eEnlarged HAADF-STEM image of the square region ind. Yellow, tangerine, and cyan dots, respectively, represent planes A, B, and C. Typical defects, including SFs and TBs are marked with orange and yellow lines, respectively.fSchematic illustration of hcp/hcp and fcc/hcp GBs in Mo2C NSs, the red dashed lines point out the irregular GBs. Along the fcc/hcp heterophase edges, both hcp phase with “ABAB” stacking and fcc phase with “ABCABC” stacking, with the coexistence of twin boundaries (TBs) and SFs are observed along the close-packed [110] f /[11 \(\overline{2}\) 0] h direction. This fcc/hcp heterophase GBs regulate the atomic arrangement of Mo 2 C lattice, which modifies the electronic structure of Mo 2 C hybrid, thus enhancing the efficiency of hydrogen production [20] . In fact, the fcc and hcp phases of Mo 2 C nanocrystals are strongly controlled by carbon activity [21] . Meanwhile, the reaction Δ H calculation clearly reveal that in anhydrous system, only the C atoms from graphene edges participate the formation of hcp Mo 2 C; while in aqueous system, carbon sources from edge and basal plane of the graphene lattice are both active and readily react with the unique Mo–O configuration to produce Mo 2 C NSs with a mixed fcc and hcp phases (Fig. 1b ). On the basis of the aforementioned characterizations, the crystalline structure of Mo 2 C NSs can be schematically illustrated in Fig. 3f , where the hcp/hcp and fcc/hcp GBs appear alternately. As a result, atomic structure analyzes clarify the atomic configuration at GBs in Mo 2 C NSs and reveal the obvious lattice distortion, accompanied by abundant atomic step edges, dislocations, TBs, and SFs, which can effectively alter the surface electronic structure. Fig. 3: Local atomic structure of GBs on Mo 2 C NSs in H-Mo 2 C/NG. a A tilted GB in Mo 2 C NS. Inset of the FFT pattern indicates a 15° misorientation between grains. a1 Enlarged HAADF-STEM image of region 1 in a . Yellow and tangerine circles represent the Mo atoms on the left and right sides of GB, respectively. a2 , a3 Enlarged HAADF-STEM images of regions 2 and 3 in a . The orange and white arrows represent SFs and displacements, respectively. b Lattice shear distortion determined from panel a , analyzed using the lattice distortion analysis (LADIA) programme. Inset is the quantitative distribution of shear strain for atoms in black-boxed region. The arrow indicates the direction of strain. The strains near GBs range from –5% to 5%. The atoms are colored according to strain scale, that is, colors for positive values represent tensile strain and those for negative values represent compressive strain. c The hcp/hcp lattices along the [1 \(\overline{2}\) 1 \(\overline{3}\) ] h /[01 \(\overline{1}\) 1] h direction, the white dashed lines point out the irregular GBs. c1 , c2 FFT patterns taken from regions 1 and 2 in c , and the corresponding projected supercell models of hcp Mo 2 C. The cyan balls represent Mo atoms. c3 , c4 Enlarged HAADF-STEM images of regions 3 and 4 in c displaying tilt GBs, step dislocations, and stepped surfaces. Step dislocations, caused by the insertion of additional planes into the otherwise self-contained lattice, highlighted with the cyan dotted box. The atomic displacement arose from this distortion at GBs is usually much greater than the relaxation displacement occurring on the crystal surface as well as the displacement caused by the coherent strain through epitaxial thin-film growth [18] . d The fcc/hcp lattices along the [110] f /[11 \(\overline{2}\) 0] h direction. The fcc/hcp GBs are marked with white solid lines. e Enlarged HAADF-STEM image of the square region in d . Yellow, tangerine, and cyan dots, respectively, represent planes A, B, and C. Typical defects, including SFs and TBs are marked with orange and yellow lines, respectively. f Schematic illustration of hcp/hcp and fcc/hcp GBs in Mo 2 C NSs, the red dashed lines point out the irregular GBs. Full size image Crystal and surface electronic structure of Mo 2 C hybrids were investigated by X-ray diffraction (XRD) and X-ray photoelectron spectroscopy (XPS) measurements. The diffraction patterns of H-Mo 2 C/NG and Mo 2 C/NG in Fig. 4a match with the hcp Mo 2 C (PDF#35-0787), which confirms the identity of Mo 2 C. Compared to Mo 2 C/NG, the diffraction peak intensity of H-Mo 2 C/NG is significantly enhanced with a narrower full width at half maxima, indicating that the introduction of water enables the epitaxial growth of Mo 2 C grains to harvest large-sized NSs [22] . No diffraction peaks of fcc Mo 2 C are detected in Mo 2 C hybrids (Supplementary Fig. 20 ), which could be attributed to the strong destruction of the periodic structure for the fcc lattice because of the alternating arrangement of fcc and hcp Mo 2 C lattices [22] . 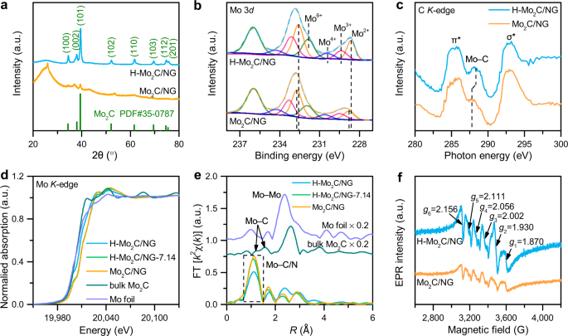Fig. 4: Spectroscopy characterization of Mo2C hybrids. aXRD patterns of H-Mo2C/NG and Mo2C/NG. The peaks near 2θ = 26° and 43° are assigned to the (002) and (100) reflections of graphene, respectively, and the weak peaks at 37° and 53° are considered to be the (\(\overline{2}\)11) and (\(\overline{2}\)22) planes of MoO2(PDF#32-0671), respectively.bThe high-resolution Mo 3dXPS spectra of H-Mo2C/NG and Mo2C/NG. Mo4+and Mo6+can be attributed to MoO2and MoO3caused by the oxidation of molybdenum species in ambient atmosphere, respectively. The Mo2+and Mo3+are assigned to carbides and nitrides, respectively, which are known to serve as active sites for HER6.cCK-edge XANES spectra of H-Mo2C/NG and Mo2C/NG. The characteristic resonances of C = C π* and C–C σ* originating from NG support.dMoK-edge XANES spectra of H-Mo2C/NG, H-Mo2C/NG-7.14, Mo2C/NG, and the reference samples. H-Mo2C/NG-7.14 and Mo2C/NG have a higher half-edge energy than that of bulk Mo2C reference, which arises from the charge-transfer from Mo to C atoms on the NG-supported Mo2C8.eMoK-edge Fourier transform EXAFS spectra of H-Mo2C/NG, H-Mo2C/NG-7.14, Mo2C/NG, and the reference samples.fEPR spectra of H-Mo2C/NG and Mo2C/NG. H-Mo2C/NG shows the EPR signals atg2= 1.930 (Mo–N species36),g1= 1.870 andg4= 2 .056 (Mo5+species37), followed byg5= 2.111 andg6= 2.156 (the resonance on conduction electrons38). Moreover, the Mo 3 d spectra of H-Mo 2 C/NG and Mo 2 C/NG are deconvoluted into four pairs of peaks (Fig. 4b ), indicating that four oxidation states for molybdenum species (+2, +3, +4, and +6) exist in Mo 2 C hybrids. Compared to Mo 2 C/NG, a negative shift of 0.17 eV is observed on Mo 2+ in H-Mo 2 C/NG, indicating the electron accumulation of Mo atoms near GBs in Mo 2 C NSs, which is beneficial to weaken the binding strength of Mo–H and thus enhance the HER activity [6] . Meanwhile, the Mo–C resonance in C K -edge X-ray absorption near-edge structure (XANES) spectra for H-Mo 2 C/NG shifts to a higher photon energy zone compared to that of Mo 2 C/NG (Fig. 4c ), which could be attributed to the enhanced orbital hybridization between the C and Mo elements, that caused by lattice distortion near GBs, facilitating electron transfer [23] . In addition, to further understand the role of water during carbonization process, a series of Mo 2 C hybrids synthesized with various water contents were also subjected to XPS measurement. As water content increases, the peak intensity of Mo–C (Supplementary Fig. 21 ) and Mo–N (Supplementary Fig. 22 ) species increases slightly, indicating that water promotes the formation of nitrogen-doped Mo 2 C. As revealed by the theoretical calculation that the reaction Δ H of TS NS to produce TS NS -N (–1.05 eV) is lower than that of TS NP to produce TS NP -N (–0.31 eV) (Supplementary Fig. 23 ), indicating that unique Mo–O configuration induced by water prefers to bind with N atoms forming Mo–N species. Fig. 4: Spectroscopy characterization of Mo 2 C hybrids. a XRD patterns of H-Mo 2 C/NG and Mo 2 C/NG. The peaks near 2θ = 26° and 43° are assigned to the (002) and (100) reflections of graphene, respectively, and the weak peaks at 37° and 53° are considered to be the ( \(\overline{2}\) 11) and ( \(\overline{2}\) 22) planes of MoO 2 (PDF#32-0671), respectively. b The high-resolution Mo 3 d XPS spectra of H-Mo 2 C/NG and Mo 2 C/NG. Mo 4+ and Mo 6+ can be attributed to MoO 2 and MoO 3 caused by the oxidation of molybdenum species in ambient atmosphere, respectively. The Mo 2+ and Mo 3+ are assigned to carbides and nitrides, respectively, which are known to serve as active sites for HER [6] . c C K -edge XANES spectra of H-Mo 2 C/NG and Mo 2 C/NG. The characteristic resonances of C = C π* and C–C σ* originating from NG support. d Mo K -edge XANES spectra of H-Mo 2 C/NG, H-Mo 2 C/NG-7.14, Mo 2 C/NG, and the reference samples. H-Mo 2 C/NG-7.14 and Mo 2 C/NG have a higher half-edge energy than that of bulk Mo 2 C reference, which arises from the charge-transfer from Mo to C atoms on the NG-supported Mo 2 C [8] . e Mo K -edge Fourier transform EXAFS spectra of H-Mo 2 C/NG, H-Mo 2 C/NG-7.14, Mo 2 C/NG, and the reference samples. f EPR spectra of H-Mo 2 C/NG and Mo 2 C/NG. H-Mo 2 C/NG shows the EPR signals at g 2 = 1.930 (Mo–N species [36] ), g 1 = 1.870 and g 4 = 2 .056 (Mo 5+ species [37] ), followed by g 5 = 2.111 and g 6 = 2.156 (the resonance on conduction electrons [38] ). Full size image To precisely probe the local coordination structure of GBs in Mo 2 C nanosheets, XANES and extended X-ray absorption fine structure (EXAFS) at Mo K-edge were conducted. Compared to H-Mo 2 C/NG-7.14 and Mo 2 C/NG, the pre-edge of H-Mo 2 C/NG obviously shifts to lower energy (Fig. 4d ), indicating the increased average electron density around Mo atoms, consistent with XPS results. The details of Mo local environment can be described through the k 2 -weighted Fourier-transformed EXAFS (FT-EXAFS) in R -space. Mo 2 C hybrids display a prominent peak at 1.30 Å originated from the Mo–C/N vector; with the increase of water content, the peak intensity of Mo–C/N path gradually decreases, indicating a low coordination number (CN) for Mo atoms in Mo 2 C (Fig. 4e ) [24] . In addition, comparing with Mo foil and bulk Mo 2 C, Mo 2 C hybrids exhibit relatively weak Mo–Mo vectors at 2.30 and 2.90 Å; these Mo–Mo paths in H-Mo 2 C/NG (2.38 and 2.95 Å) are slightly stretched compared to H-Mo 2 C/NG-7.14 (2.29 and 2.87 Å) and Mo 2 C/NG (2.29 and 2.87 Å). These results indicate that numerous Mo atoms in H-Mo 2 C/NG are misplaced and deviated from the normal crystalline position, which could be attributed to the high-angle GBs with large lattice strain in Mo 2 C NSs [25] . 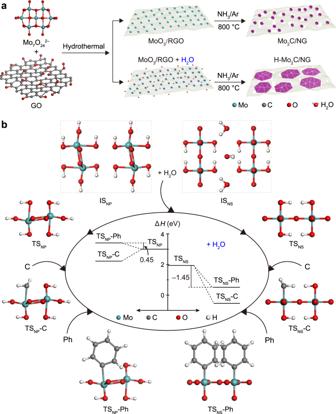Furthermore, quantitative EXAFS fitting was performed using DFT optimized hcp Mo 2 C structure to extract the structural parameters, and the fitting results are displayed in Supplementary Fig. 24 . Fig. 1: Formation of H-Mo2C/NG. aSchematic diagram of the synthesis of Mo2C/NG and H-Mo2C/NG.bVarious reaction states of ISNPand ISNSalong the reaction pathway. Inset shows the corresponding reaction ΔHdiagram. The reaction ΔHfor TSNSconversion to TSNS-C (–2.48 eV) is lower than that of TSNPconversion to TSNP-C (–0.73 eV), indicating that water promotes the formation of Mo2C during carbonization process. Briefly, compared to H-Mo 2 C/NG-7.14 and Mo 2 C/NG, H-Mo 2 C/NG has two different Mo–C/N paths and low CN (Supplementary Table 1 ), highlighting the structural distortion and carbon defects, which further confirms the construction of GBs in Mo 2 C NSs. Moreover, the surface defects in Mo 2 C NSs are further resolved with the electron paramagnetic resonance (EPR) spectroscopy. As illustrated in Fig. 4f , the EPR signal at g 3 = 2.002 for H-Mo 2 C/NG is attributed to the unpaired electrons trapped on carbon defects at Mo 2 C GBs; [26] where a slightly lower signal is observed for Mo 2 C/NG, demonstrating relatively high concentration of coordination unsaturated Mo atoms in Mo 2 C NSs, consistent with EXAFS results. The above results demonstrate that the water-assisted carbothermal reaction strategy successfully constructs ultrathin Mo 2 C NSs with high-density GBs anchored on NG support, which provides sufficient active sites and the possibility of modulating the interface atomic and electronic configurations. Electrocatalytic HER performance The catalytic performance of Mo 2 C hybrids was investigated by a three-electrode system in 0.5 M H 2 SO 4 and 1.0 M KOH solutions (see more details in Methods). As revealed in Fig. 5a , H-Mo 2 C/NG shows the highest HER performance among all catalysts in acidic media, and only requires an overpotential of 10 mV to achieve the geometric current density of –10 mA cm –2 ( η 10 ), significantly superior to the Mo 2 C/NG ( η 10 = 138 mV) and even Pt/C catalyst ( η 10 = 19 mV). 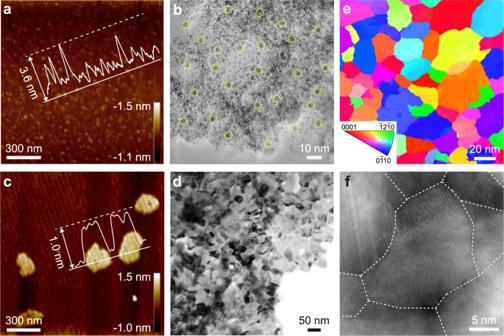Furthermore, the Tafel slope of H-Mo 2 C/NG is 38 mV dec –1 (Fig. 5b ), which far surpasses that of Mo 2 C/NG (137 mV dec –1 ) and is even comparable to that of state-of-the-art Pt/C catalyst (34 mV dec –1 ), suggesting that H-Mo 2 C/NG possesses more fast kinetics with the Heyrovsky reaction as the rate-determining step [18] . Fig. 2: Structural characterization of Mo2C hybrids. a,cAFM images ofaMo2C/NG andcH-Mo2C/NG and their corresponding height profiles.b,dTEM images ofbMo2C/NG anddH-Mo2C/NG. Mo2C NPs are highlighted by yellow dotted circles.eInverse pole figure (IPF) images from PED analysis of H-Mo2C/NG.fRepresentative HADDF-STEM image of H-Mo2C/NG, the dashed lines point out the irregular GBs. The exchange current density ( j 0 ) of H-Mo 2 C/NG is calculated to be 5.47 mA cm −2 , which is much higher than that of Mo 2 C/NG (0.80 mA cm −2 ) (Supplementary Table 2 ), further underscoring favorable HER kinetics. Meanwhile, H-Mo 2 C/NG also demonstrates promising HER activity in alkaline media. H-Mo 2 C/NG merely requires overpotentials of 63 and 163 mV to reach –10 and –100 mA cm –2 , respectively, which are comparable to commercial Pt/C catalyst ( η 10 : 57 mV and η 100 : 173 mV) and significantly better than those of Mo 2 C/NG ( η 10 : 107 mV and η 100 : 388 mV) (Fig. 5c ). Compared to Mo 2 C/NG catalyst, H-Mo 2 C/NG also affords a lower Tafel slope of 48 mV dec –1 (Fig. 5d ) and higher j 0 value (0.75 mA cm –2 ), which reveals the same favorable HER kinetics as in acidic media for H-Mo 2 C/NG. To further study the effect of GBs on HER activity, we performed electrocatalytic hydrogen evolution tests on a series of Mo 2 C hybrids. Obviously, as the water content increases, the η 10 and Tafel slopes on Mo 2 C hybrids firstly decrease and then increase (Supplementary Figs. 25 - 28 ), where H-Mo 2 C/NG with the highest GB density achieves the best HER performance. These results suggest that the GBs in Mo 2 C NSs can effectively enhance the intrinsic HER activity of the Mo 2 C hybrids. Additionally, to gain insight into the superior catalytic activity of H-Mo 2 C/NG, the turnover frequency (TOF) was calculated (Supplementary Fig. 29 and Supplementary Note 4 ). As displayed in Fig. 5e , H-Mo 2 C/NG affords the TOF values of 21.33 and 3.81 H 2 s –1 at η = 100 mV in acidic and alkaline electrolytes, respectively, which are quite larger than those of Mo 2 C/NG (0.57 and 1.08 H 2 s –1 ), as well as other control samples (Supplementary Fig. 30 ), confirming the high HER activity of H-Mo 2 C/NG. To further identify the intrinsic activity of H-Mo 2 C/NG, geometric current density ( j ) was normalized by electrochemical active surface area (ECSA; j ECSA ), which was determined by deriving the electrochemical double-layer capacitance ( C dl ). The C dl of H-Mo 2 C/NG (23.8 mF cm –2 ) is slightly higher than that of Mo 2 C/NG (19.7 mF cm –2 ), suggesting the close ECSA values (Fig. 5f and Supplementary Note 5 ). Yet, H-Mo 2 C/NG delivers the j ECSA values of 109.53 and 10.57 μA cm –2 at η = 50 mV in 0.5 M H 2 SO 4 and 1.0 M KOH (Supplementary Figs. 31 , 32 ), which are evidently higher than those of Mo 2 C/NG (3.70 and 6.23 μA cm –2 ) and Pt/C (80.16 and 9.86 μA cm –2 ), respectively, revealing better intrinsic HER activity of H-Mo 2 C/NG with massive GBs, even outperforming benchmark Pt/C catalyst. In comparison with non-precious metal HER electrocatalysts reported recently (Supplementary Tables 3 , 4 ), H-Mo 2 C/NG exhibits almost the lowest overpotential and Tafel slope, illustrating the super HER activity in pH-universal electrolyte. Besides, H-Mo 2 C/NG has a small charge-transfer resistance ( R ct ) (2.5 and 2.1 Ω) in 0.5 M H 2 SO 4 and 1.0 M KOH, respectively, which is much lower than those of Mo 2 C/NG (5.5 and 12.5 Ω) and other control samples (Supplementary Fig. 33 ). This result indicates that H-Mo 2 C/NG possesses much fast electron transfer kinetics during HER process, which is attributed to the unique structure of Mo 2 C NSs with chemically connected GBs, shortening the electron transfer pathway between active sites [27] . Fig. 5: HER performance. a , c The polarization curves and b , d the relevant Tafel plots of H-Mo 2 C/NG, Mo 2 C/NG, and Pt/C in a , b 0.5 M H 2 SO 4 and c , d 1.0 M KOH, respectively. e TOF values of H-Mo 2 C/NG and Mo 2 C/NG in 0.5 M H 2 SO 4 and 1.0 M KOH. f The plots of the current density versus the scan rate for H-Mo 2 C/NG and Mo 2 C/NG in 1.0 M KOH. Inset is cyclic voltammetry (CV) cycles of H-Mo 2 C/NG. g Galvanostatic measurement of H-Mo 2 C/NG in 0.5 M H 2 SO 4 and 1.0 M KOH at j = –100, –200, and –300 mA cm –2 , respectively. Full size image For real applications, the stability and durability of H-Mo 2 C/NG were further analyzed. As illustrated in Supplementary Fig. 34 , after 10,000 or even 50,000 cycles in 0.5 M H 2 SO 4 and 1.0 M KOH, the shifts of polarization curves for H-Mo 2 C/NG are negligible compared with the initial curves. Meanwhile, we performed aggressive long-term stability examine on H-Mo 2 C/NG by continuous galvanostatic measurement (Fig. 5g ). After 100,000 s of operation at j = −100, −200, and −300 mA cm −2 , the potentials of H-Mo 2 C/NG only increase by 8, 14, and 38 mV in 0.5 M H 2 SO 4 , and 11, 13, and 36 mV in 1.0 M KOH, respectively. In contrast, the potentials of Pt/C catalyst at j = −200 mA cm −2 increase by 136 and 110 mV in 0.5 M H 2 SO 4 and 1.0 M KOH, respectively. In addition, TEM characterization shows that Mo 2 C nanocrystals in H-Mo 2 C/NG still maintain an ultrathin nanosheet structure with highly exposed high-density GBs after electrochemical cycling (Supplementary Fig. 35 ). XRD characterization displays that Mo 2 C is well crystallized, and no other phase is experimentally detected (Supplementary Fig. 36 ). The chemical valence state of Mo species remains almost unchanged, further indicating the robustness of H-Mo 2 C/NG in the electrocatalytic HER process (Supplementary Fig. 37 ). It should be noted that most synthesized 2D Mo 2 C catalysts cannot withstand a high current density and operate for a long-lasting lifetime in a wide pH range because of the weak interfacial adhesion with adjacent nanocrystals or substrates [11] , [13] . In this work, the excellent physicochemical stability of H-Mo 2 C/NG can be attributed to the chemical connection of Mo 2 C GBs and strong interaction of Mo 2 C NSs with NG sheets through Mo–C bonds. Moreover, the general synthetic strategy of GB-rich NSs can also be extended to other transition metal carbide systems (Supplementary Fig. 38 ), such as vanadium (Supplementary Fig. 39 ), niobium (Supplementary Fig. 40 ), tantalum (Supplementary Fig. 41 ), and tungsten (Supplementary Fig. 42 ), and yield excellent HER performances in pH-universal electrolyte (Supplementary Fig. 43 ), demonstrating the generality of this method, which provides an alternative way to develop high-efficiency catalysts through GB engineering. DFT calculations To understand the correlation between the electronic structure and catalytic performance in GB-rich Mo 2 C plane, DFT calculations were conducted. According to the HAADF-STEM images of Mo 2 C NSs (Fig. 3 and Supplementary Figs. 16 , 19 ), the computational models of fcc/hcp, fcc/fcc, and hcp/hcp GBs were constructed, respectively. The DFT calculation shows that the fcc/hcp Mo 2 C slab surface exists various kinds of trigonal pyramid-like structures (Supplementary Fig. 44 ), in which Mo atom locates at top and pyramidally coordinates with three C atoms at bottom, forming a typical trigonal pyramid (MoC 3 ) configuration (Fig. 6a ). Depending on the height of the pyramid-shaped MoC 3 skeleton on the fcc/hcp Mo 2 C superlattice surface, the corresponding configuration of MoC 3 can be schematically classified into three types: (i) approximative triangular plane (S1), (ii) intermediate height (S2), and (iii) high height (S3). The hcp Mo 2 C surface consists of S1 and S3 structures, in which the S3 structure typically represents common bulk Mo 2 C configuration and is predominant; on the fcc Mo 2 C surface, MoC 3 pyramids only present S3 structure. Notably, the fcc region of the fcc/hcp GB is contracted interface with a smaller Mo–Mo distance corresponding to the S3 structure. While the hcp region of the fcc/hcp GB exhibits an elongated interface with a larger Mo–Mo distance, where MoC 3 pyramids at GB have a medium height and belong to S2 structure. Fig. 6: Relationship between HER activity and the d z 2 orbital energy level. a Structural models and relevant electronic states of Mo d orbital for MoC 3 configurations. S1: MoC 3 triangular plane, S2: intermediate height, S3: high height. PDOS of Mo d orbital for b S2 and c S3 structures. d Schematic diagram of hybridization of H 1 s orbital and Mo d z 2 orbital. e Correlation of the Mo d z 2 orbital energy level and H ads , inset is the corresponding fitting equation. Full size image Furthermore, to find the rule for the GB effect on HER electrocatalysis, the crystal field analyzes of MoC 3 pyramids for S2 and S3 structures were performed with the projected density of state (PDOS) calculation, as illustrated in Fig. 6b and c , respectively. Evidently, with the increase of the height (from bottom C 3 plane to atop Mo atom), the energy level of the Mo d z 2 orbital also increases correspondingly. Consequently, these three low-lying orbitals further undergo symmetry breaking, rising the Mo d z 2 orbital state into distinct energy levels [28] (Fig. 6a ). In the electrocatalytic HER process, the adsorption of H atoms on the Mo atoms forms σ bonds, which originate from the orbital hybridization between the H 1 s orbitals and the Mo d z 2 orbitals (Fig. 6d ). According to the Sabatier principle, the ideal electrocatalyst should bind H intermediate neither too strongly nor too weakly [29] . Therefore, the optimized adsorption free energy and fast HER kinetics can be achieved by manipulating the bond strength between the H 1 s orbital and Mo d z 2 orbital [4] . The bond strength is defined as: 
    E∝f(S,E_d_z^2)/E_s-E_d_z^2
 (1) Where E s and \({E}_{{{\rm{d}}}_{{z}^{2}}}\) are the energy levels of H 1 s orbital and Mo d z 2 orbital, respectively. S is orbit overlap population of H 1 s orbital and Mo d z 2 orbital. Within these contexts, we calculated the H adsorption free energy ( H ads ) of surface Mo atoms on the model of fcc/hcp GB, and studied its relationship with the Mo d z 2 orbital energy level (Fig. 6e ). Where the numerical fitting over the calculated H ads and the Mo d z 2 orbital energy level follows the similar function as the Eq. ( 1 ) of bond strength, that is, the adsorption energy varies with the Mo d z 2 orbital energy level. As a result, the intrinsic HER activity exhibits a strong dependence on the Mo d z 2 orbital energy level, which rationalizes the role of d z 2 orbital energy level as one of the most important activity descriptors for HER in Mo 2 C systems. Compared with the state-of-the-art descriptors such as band-energy theory and work function that describe the properties of the whole surface [30] , the d z 2 orbital energy level is more relevant to the active site of the catalysts. Therefore, the descriptor d z 2 orbital energy level could be used as a figure of merit for designing transition metal catalyst with well-defined active sites for electrocatalytic HER reaction. Additionally, the H ads on the Mo atoms near the fcc/fcc and hcp/hcp homophase Mo 2 C GBs also display close-to-zero values, such as –0.044, 0.035, and 0.038 eV (Supplementary Figs. 45 and 46 ), which also contribute to the excellent HER activity. As a result, the DFT results confirm that GBs in ultrathin Mo 2 C NSs can significantly alter the electronic structures of H-Mo 2 C/NG electrocatalyst, and the intrinsic HER activity strongly depends on the Mo d z 2 orbital energy level controlled by the MoC 3 pyramid configuration. In summary, ultrathin Mo 2 C NSs with rich GBs supported on NG have been developed by facile hydrothermal and water-assisted carbothermal reactions with GO as carbon source. During carbonization process, water induces structural evolution of Mo 2 C nanocrystals from NPs to NSs and controls the GB density of Mo 2 C NSs as well. In H-Mo 2 C/NG, the dense polycrystalline Mo 2 C NSs with massive irregular GBs are chemically connected to NG through Mo–C bonds, which afford ultra-high fraction of active sites for electrolysis, exhibiting high reproducibility in terms of structure and performance. The inherent HER activity of H-Mo 2 C/NG electrocatalyst strongly depends on the d z 2 orbital energy level of Mo atoms, which is controlled by the MoC 3 pyramid configuration. This work provides a horizon for rationally designing GB interfaces of transition metal electrocatalysts to achieve excellent HER activities, and establishes a descriptor of the d z 2 orbital energy level for the design of high-performance catalysts. Chemicals All chemicals were purchased from commercial sources (Sigma Aldrich, Energy Chemical) without further purification. GO was synthesized from graphite flakes by the improved Hummers method [31] . Synthesis of H-Mo 2 C/NG First, the GO suspension was prepared by adding 0.16 g GO into 80 mL deionized water and sonicating for 10 h. Typically, 0.4470 g (NH 4 ) 6 Mo 7 O 24 ·4H 2 O were added into the GO suspension and sonicated for another 4 h. Subsequently, above mixture was transferred to a Teflon-lined autoclave and heated at 190 °C for 12 h to harvest MoO 3 /RGO intermediate. Next, the MoO 3 /RGO intermediate was freeze-dried to obtain sponge columns with various water contents, including 0, 0.41, 7.14, 13.52, 18.56, 30.98, and 43.28 wt%. The MoO 3 /RGO with various water contents were put into a tubular quartz furnace for heat treatment. After pumping and purging the system with Ar for 30 min, the temperature was ramped at 10 °C min −1 up to 800 °C with the feeding of Ar (150 sccm) and NH 3 (100 sccm). The reaction was allowed to proceed for 3 h and the final product was fast cooled to room temperature by quickly removing the sample from the hot zone of the furnace under the protection of flowing Ar. The final catalysts were named H-Mo 2 C/NG-X, where X was the water content retained in MoO 3 /RGO intermediate, for example, H-Mo 2 C/NG-7.14 (the water content was 7.14 wt%). In our report, H-Mo 2 C/NG-18.56 and H-Mo 2 C/NG-0 were denoted as H-Mo 2 C/NG and Mo 2 C/NG unless otherwise specified, respectively. Material characterization Morphological structure characterizations of Mo 2 C hybrids were performed on SEM (JEOL-JSM-7001F) and TEM (FEI Talos F200X, FEI Titan ChemisSTEM, FEI Titan Themis). HAADF-STEM images were carried out by a Cs-corrected FEI Titan G2 60-300 equipped with a Super-X EDS detector. The LADIA package was used to analysis the strain states of Mo 2 C nanocrystals during the loading and unloading of tensile stress [32] . The surface electronic structure was checked by XPS spectra (XPX, PHI-5702). The C and N K-edge NEXAFS spectra were measured at the photoemission end-station at beamline BL10B in the National Synchrotron Radiation Laboratory (NSRL) in Hefei, China. X-ray absorption spectra (XANES and EXAFS) of Mo K-edge were measured on VESPERS beamline at the Canadian Light Source, by scanning a double crystal Si (111) monochromator and collecting emitted X-ray fluorescence. Electrochemical measurements Electrochemical measurements were conducted on a typical three-electrode system (CH Instruments 760E). All potentials were referenced to a reversible hydrogen electrode (RHE) and without iR compensation. The binder solution was prepared by mixing of 5 wt% Nafion solution (40 μL) with 1 mL of 4:1 v/v deionized water/ethanol. 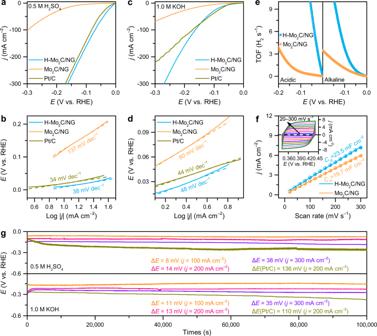Fig. 5: HER performance. a,cThe polarization curves andb,dthe relevant Tafel plots of H-Mo2C/NG, Mo2C/NG, and Pt/C ina,b0.5 M H2SO4andc,d1.0 M KOH, respectively.eTOF values of H-Mo2C/NG and Mo2C/NG in 0.5 M H2SO4and 1.0 M KOH.fThe plots of the current density versus the scan rate for H-Mo2C/NG and Mo2C/NG in 1.0 M KOH. Inset is cyclic voltammetry (CV) cycles of H-Mo2C/NG.gGalvanostatic measurement of H-Mo2C/NG in 0.5 M H2SO4and 1.0 M KOH atj= –100, –200, and –300 mA cm–2, respectively. 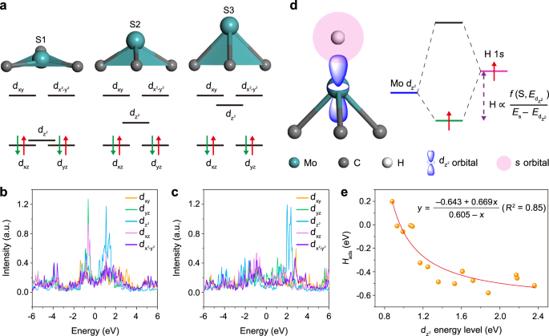Fig. 6: Relationship between HER activity and thedz2orbital energy level. aStructural models and relevant electronic states of Modorbital for MoC3configurations. S1: MoC3triangular plane, S2: intermediate height, S3: high height. PDOS of Modorbital forbS2 andcS3 structures.dSchematic diagram of hybridization of H 1sorbital and Modz2orbital.eCorrelation of the Modz2orbital energy level andHads, inset is the corresponding fitting equation. The catalyst ink was then prepared by dispersion of 2 mg Mo 2 C hybrids (H-Mo 2 C/NG, Mo 2 C/NG, and control samples) into binder solution followed by ultrasonication for 2 h. In Mo 2 C hybrids, molybdenum atoms are the active species, and molybdenum loading (~ 8 wt%, Supplementary Table 5 ) is basically the same. To maintain the same metal load, 8 mg Pt/C catalyst (20 wt% Pt on graphitized carbon, Johnson Matthey) ink was prepared in the same way. The ink (10 μL) was then dripped onto a carbon fiber paper (CFP, 5 mm × 5 mm) as the working electrode. The electrode was allowed to dry at room temperature for at least 24 h before measurement. After drying, a catalyst (Mo 2 C hybrids and Pt/C) mass loading of 0.038 mg cm –2 was obtained. A graphite rod as the counter electrode and saturated calomel electrode (SCE) as the reference electrode. All potentials were referenced to RHE: E RHE = E SCE + (0.242 + 0.059 pH) V. In 0.5 M H 2 SO 4 and 1.0 M KOH solutions, the polarization curves were obtained at the electrode potential of 0 to 0.45 V using a scan rate of 50 mV s −1 . The electrochemical EIS was performed from 10 –2 to 10 6 Hz with an AC voltage of –5 mV. Galvanostatic charge discharge curves of H-Mo 2 C/NG were recorded at j = –100, –200, and –300 mA cm –2 . Prior to all measurements, the electrochemical system was purged with H 2 bubbles for 30 min, and then conducted all electrochemical measurements at room temperature (25 °C) under ambient atmosphere. DFT calculations The first-principles calculations based on the DFT were performed within generalized gradient approximation (GGA). Core electron states were represented by the projector augmented-wave method as implemented in the Vienna ab initio simulation package (VASP) [33] , [34] . The Perdew–Burke–Ernzerhof exchange-correlation functional and a plane wave representation for the wave function with a cut-off energy of 450 eV were used [35] , more details can be found in Supporting Information (Supplementary Note 6 ). The atomic coordinates of the H adsorption on the fcc/hcp GB model to generate Fig. 6e are listed in VASP CONTCAR format (Supplementary Data 1 ).